Quality control of protein reagents for the improvement of research data reproducibility (1) For recombinant proteins, the complete sequence of the construct used in the reported experiments should be made available and we highly recommend confirming the sequence after cloning by sequencing to avoid wasteful production trials. (2) Expression, purification and storage conditions should be fully described such that they may be accurately reproduced in any laboratory. (3) The method used for measuring the protein concentration should be given (1) Protein purity should be assessed by any of common techniques such as SDS-PAGE, Capillary Electrophoresis (CE), Reversed Phase Liquid Chromatography (RPLC). Mass Spectrometry (MS) and RPLC help to detect the presence of contaminating proteins, sample proteolysis and minor truncations. (2) Homogeneity/dispersity refers here to the size distribution of the protein sample, which can generally be correlated with oligomeric state (monomer, dimer etc.) or the presence of aggregates. Whereas poly-dispersity is not per se an indication of instability, preparations showing the presence of ‘incorrect’ oligomeric states or higher order ‘aggregates’ suggest that the protein may not be in an optimal/functional state. This can have a dramatic effect on the results of experiments to determine e.g. enzyme kinetics and protein-ligand interactions, essentially as a result of an overestimation of the concentration of active protein. Protein homogeneity/dispersity may be assessed by Dynamic Light Scattering (DLS), size exclusion chromatography (SEC) or, preferably, by SEC coupled to multi-angle light scattering. (3) The identity of a sample can be confirmed using either ‘bottom-up’ MS (mass fingerprinting or tryptic digests) or ‘top-down’ MS (by measuring intact protein mass). The former will confirm that the correct protein is being used and not e.g. a host protein of similar mass that has been purified in error. The latter will confirm the identity of the protein and will also indicate whether it has suffered any proteolysis during purification (intactness/micro-heterogeneity). In addition to this short list of minimal/essential controls, other techniques are recommended to further characterize protein samples and their suitability as experimental reagents, for instance the folding state of proteins and the specific activity of enzymes. Proteins produced in Escherichia coli that are destined for use in experiments with cultured cells should be tested for the presence of lipopolysaccharides/endotoxins and UV spectrophotometry is mandatory for DNA/RNA binding proteins. Examples in which protein quality assessment resulted in improvements of sample quality with critical impact on downstream experimental results are presented in supplementary information (Supplementary Note 2 , Supplementary Figs. 8 – 12 ). The results of a large scale survey among users who volunteered applying the guidelines in their routine experiments has also been carried out [15] . In our experience, the application of the limited number of simple QC tests suggested above provides reliable indicators of the quality of the protein employed as experimental reagents, and yields more reproducible results in downstream applications. We believe that their implementation and the public availability of such QC data could therefore significantly increase the level of confidence in the published data resulting from the use of protein reagents, as well as the ability to reliably reproduce the experimental data. This condition, which should ideally be the norm, is in reality challenged by several factors as reported in a recent survey [5] . Selective reporting, insufficient availability of raw data and the paucity of information in many ‘Materials and Methods’ sections are all factors which contribute to create opacity. The decline of the essential materials and methods sections of published papers dates back, understandably, to the times when many journals were available only in print and the pressures to minimize the sizes of submitted papers. With the advent of on-line publishing it is time to advocate the (re-) integration of these essential sections to their former status to allow other researchers to reproduce the data therein without resorting to making contact with the authors. Although this effect has been partly mitigated by the current availability of Supplementary Data sections in many on-line journals, the presented data often falls short of a full description of the experimental conditions used and often lacks any form of QC data relating to protein quality. The present interest of Editors for the systematic storage of (raw) data [ https://www.springernature.com/gp/open-research/open-data/practical-challenges-white-paper ] should consider also the inclusion of this methodological data. We suggest that implementation of guidelines for protein quality evaluation should be considered an entry point towards the development of improved and ideally compulsory reporting practices of data obtained with protein reagents. It is our contention that ‘Supplementary Data’ sections should also contain details of the QC tests performed on any protein/peptide reagents used in a study, independent of the source of the protein reagent (commercial vendors or purified in an academic lab), in order to give referees and readers an indication of the quality of the materials being used to derive any given data set. To this effect, we suggest the development—in co-operation with journal editors—of a standardized form for QC reporting and annotation for authors to complete during the submission process. 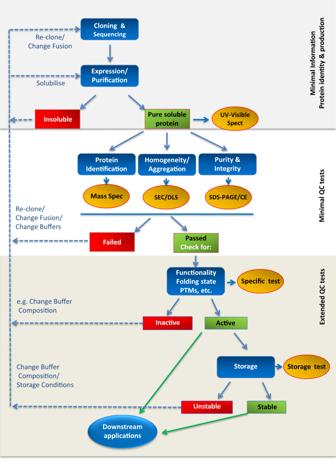Fig. 1: Protein reagents: evaluation of Protein Identity, Preparation and Quality Control. Blue icons indicate process steps, whereas yellow icons display quality control requested experiments. The actual DNA sequence of the clone must be verified for its identity/correctness (correspondence to original clone, no mutations) before starting its expression. Following purification, the identity of the protein must be confirmed (by Mass Spectrometry), its purity and integrity evaluated (SDS-PAGE/CE), and its homogeneity (i.e., size distribution/aggregation state) checked to assess size distribution (i.e., monodispersity/polydispersity). The most accessible tests are reported (SEC, DLS), alternatives can be found in the guidelines. If all minimal QC tests are passed, proteins should be tested for further properties, e.g. their functionality or their folding state before being used as reagents. Further analyses are necessary for specific protein applications, as it can be the case of DNA contaminations (extended tests described in the on-line guidelines/SN1), and to evaluate the possibility to store the protein. If proteins do not pass any of the check steps, their production/storage process should be optimized. Summarizing, the minimum QC relies on three parameters (i.e., identity, purity, integrity and homogeneity) requiring three (first-line) analytical methods only. As indicated, it is possible to choose between alternatives: SDS-PAGE or CE, analytical SEC or DLS. The requirement in terms of protein is roughly 100 μg [SDS-PAGE, 10 μg (Coomassie blue staining); Mass Spectrometry, 60 μg; Analytical SEC, 30 μg (for Dynamic Light Scattering, 20 μg, the sample can be recovered)]. UV-Visible spectrophotometry is advised since the protein is recycled and several pieces of information can be rapidly collected (Supplementary Note1). A model of such a checklist is illustrated in Supplementary Table 1 and could be made available to referees and editors but also published in the supplementary material to allow reader scrutiny. Finally, all the stakeholders—scientists, editors and funding agencies—will profit from improving data reliability and reproduction by means of systematic and accurate reagent QC. Such practices should minimize the wasteing of time and resources and, in addition, favor future metadata analysis.